An evolutionarily conserved three-dimensional structure in the vertebrateIrxclusters facilitates enhancer sharing and coregulation Developmental gene clusters are paradigms for the study of gene regulation; however, the mechanisms that mediate phenomena such as coregulation and enhancer sharing remain largely elusive. Here we address this issue by analysing the vertebrate Irx clusters. We first present a deep enhancer screen of a 2-Mbp span covering the IrxA cluster. Using chromosome conformation capture, we show that enhancer sharing is widespread within the cluster, explaining its evolutionarily conserved organization. We also identify a three-dimensional architecture, probably formed through interactions with CCCTC-binding factor, which is present within both Irx clusters of mouse, Xenopus and zebrafish. This architecture brings the promoters of the first two genes together in the same chromatin landscape. We propose that this unique and evolutionarily conserved genomic architecture of the vertebrate Irx clusters is essential for the coregulation of the first two genes and simultaneously maintains the third gene in a partially independent regulatory landscape. The Iroquois ( Irx/iro ) genes, present in all metazoans, encode TALE class homeoproteins that exert multiple functions during animal development (reviewed in ref. 1 ). One of the striking characteristics of the members of this gene family is their organization in large genomic clusters, which have arisen independently across the animal kingdom [2] , [3] , [4] , [5] , [6] . In these clusters, the Irx genes are separated by large intergenic regions, denoted gene deserts. Most vertebrates contain six Irx genes grouped in two paralog clusters of three genes each [2] , [3] . The IrxA cluster contains Irx1 , Irx2 and Irx4 , and the IrxB cluster contains Irx3 , Irx5 and Irx6 . In all vertebrates analysed, the Irx1/Irx2 and Irx3/Irx5 pairs have very similar expression patterns [3] , [7] , [8] , [9] , [10] , [11] , [12] , [13] , [14] . The expression of the third gene in each cluster, Irx4 or Irx6 , is usually more divergent. However, in some tissues, all the genes of a cluster, or even of both clusters, are identically expressed [3] , [7] , [10] , [14] . Why these genes tend to be organized in such large clusters remains a mystery. One possibility is that the different genes within a cluster share conserved intergenic regulatory elements. Consistent with this idea, we have identified many highly conserved non-coding regions (HCNRs) that function as cis -regulatory elements and are distributed throughout the gene deserts of the IrxB cluster [3] . These regulatory sequences drive the expression in sub-domains of the territories expressing the IrxB genes. Many of these sub-domains show expression of more than one IrxB gene, pointing again to the presence of shared enhancers. However, to date there has been no reported genetic or molecular evidence that enhancer sharing exists within vertebrate Irx clusters. Here we present an extensive enhancer screen of the IrxA cluster. We demonstrate the presence of multiple cis -regulatory elements throughout this genomic region, which promote expression in sub-domains of the IrxA -expressing territories. Moreover, using the chromosome conformation capture (3C) technology, a PCR-based method that allows determining the physical in vivo interaction between any chromatin segments (reviewed in ref. 15 ), we examined the interaction of four representative enhancers with the promoters of the three IrxA genes. We show that enhancers are shared among the Irx promoters, although they preferentially interact with the first two genes of the cluster. This provides direct physical evidence that enhancers are shared in the cluster, probably placing a strong evolutionary constraint that maintains the linear association of these genes. Most interestingly, we also identify an evolutionarily conserved three-dimensional (3D) architecture, present in both Irx clusters of all vertebrates, that brings the Irx1/3 and Irx2/5 promoters into physical contact. This loop might explain the preferential interaction of the various enhancers with the first two genes of the IrxA cluster and the coregulation of these genes in both clusters. We finally show that the formation of this evolutionarily conserved loop in vertebrates is probably mediated by CCCTC-binding factor (CTCF). Our work not only provides the first demonstration that enhancers are shared within the Irx clusters, but also identifies a deeply conserved three-dimensional architecture that predates cluster duplication. This architecture would help to generate different regulatory landscapes for linearly arranged genes. Cis -regulatory landscape of the IrxA cluster Many reports have shown that HCNRs are enriched in cis -regulatory elements (see for example refs 3 , 16 , 17 ). To gain insight into the regulatory landscape of the IrxA cluster in vertebrates, we used an in vivo transgenic assay to examine the activity of 88 HCNRs distributed throughout the cluster and present in all tetrapods. These regions were amplified from Xenopus tropicalis genomic DNA and cloned in an appropriate vector for Xenopus transgenesis (see Methods). Of the 88 HCNRs, 16 (18%) activated expression in a robust and reproducible manner at the tail-bud stage ( Fig. 1 ), a proportion in line with our previous analysis of HCNRs from the IrxB cluster [3] . These HCNRs drove reporter expression within sub-domains of the endogenous pattern of IrxA genes at this stage [14] , such as the midbrain, hindbrain, spinal cord, kidney and otic vesicle ( Fig. 1 ). These patterns are discrete and restricted to specific territories, although the domains of several elements partially overlap. 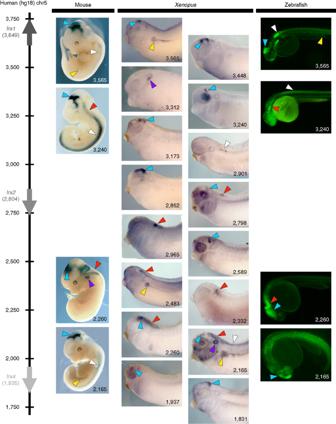Figure 1: Multiple enhancers are distributed along the theIrxAcluster. The black vertical line at the left depicts theIrxAcluster, showing coordinates (kbp) of human chromosome 5. Columns show enhancer activity of different HCNRs in embryos of mouse (stage E11.5),Xenopus(stage 30) and zebrafish (24–36 h.p.f.). Enhancers are named according to the coordinates (in kilobases) of their human HCNR counteparts. Orthologous regions promote expression in largely equivalent territories. Arrowheads mark tissues by colour as follows: blue, midbrain; red, hindbrain; white, spinal cord; yellow, kidney; and purple, otic vesicle. Figure 1: Multiple enhancers are distributed along the the IrxA cluster. The black vertical line at the left depicts the IrxA cluster, showing coordinates (kbp) of human chromosome 5. Columns show enhancer activity of different HCNRs in embryos of mouse (stage E11.5), Xenopus (stage 30) and zebrafish (24–36 h.p.f.). Enhancers are named according to the coordinates (in kilobases) of their human HCNR counteparts. Orthologous regions promote expression in largely equivalent territories. Arrowheads mark tissues by colour as follows: blue, midbrain; red, hindbrain; white, spinal cord; yellow, kidney; and purple, otic vesicle. Full size image Eight of the IrxA HCNRs are partially conserved in the IrxB cluster in largely equivalent genomic locations [18] indicating an origin that predates the duplication of the clusters. Interestingly, of these eight paralogous sequences, five were positive in our Xenopus transgenic assay (2,165, 2,695, 3,173, 3,240 and 3,565) and all IrxA and IrxB paralogues show similar regulatory activities, with the exception of the paralogue region of 3,240 which showed no enhancer activity ( Supplementary Fig. S1 and see ref. 3 ). To test the evolutionary conservation of enhancer function in vertebrates, we next examined the activity of four of these HCNRs in mouse and zebrafish transgenic assays. In most cases, these orthologous regions activated the expression of reporter genes in territories largely equivalent to those promoted by the Xenopus HCNRs ( Fig. 1 ). IrxA enhancers interact with multiple Irx promoters Most enhancers identified in this study drive expression in territories expressing more than one Irx gene, making it likely that their regulatory activity is shared by different genes of the cluster. To explore this, we examined physical interactions in vivo between different regulatory elements and the three Irx promoters by means of 3C [19] . For these experiments, we selected four enhancers well distributed along the cluster, two located between the Irx1 and Irx2 genes (3,565 and 3,240, Figs 1 and 2a ) and the other two located in the Irx2 / Irx4 intergenic region (2,260 and 2,165, Figs 1 and 2a ). Of these four enhancers, two are conserved in both Irx clusters (3,565 and 2,165) and the other two are specific for the IrxA cluster (3,240 and 2,260). Moreover, as for our 3C experiments we used tissues dissected from embryos, to increase homogeneity, we selected enhancers driving strong expression in as many cells as possible. The enhancers were taken as fixed positions, and interactions were tested with each promoter and two flanking regions ∼ 30 kbp upstream and downstream. As we observed a clear inverse relationship between distance and interaction level, we defined the average of the interactions of each enhancer with its two promoter-flanking regions as the background level of interaction (see Fig. 2b ). These enhancer–promoter interactions were examined in midbrain–hindbrain and limb tissues. As all four enhancers are predominantly active in the neuroectoderm ( Figs 1 and 2a ), we expected that any enhancer–promoter interactions would be stronger in neural tissues than in limb tissues. This was indeed the case, and all enhancers seem to interact preferentially with Irx promoters rather than with the neighbouring chromatin region, this interaction being stronger in neural tissue ( Fig. 2b ). Several enhancers show significant interaction with more than one promoter (3,565 with Irx1 and Irx4 ; 3,240 with Irx1 and Irx2 ), and these enhancer–promoter interactions can occur even over unprecedentedly long distances of 1.5 Mbp (3,565 with Irx4 and 2,260 with Irx1 ). It is also noteworthy that most enhancers interact preferentially with the first two genes of the cluster, which raises the question of what molecular mechanism underlies such preferential interaction. 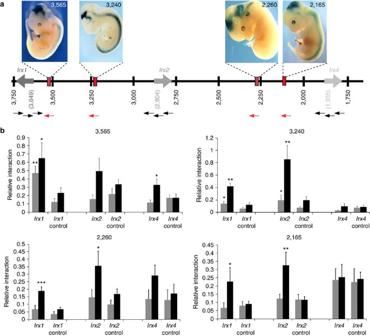Figure 2: Enhancers physically interact with multipleIrxpromoters. (a) Expression patterns of the enhancers tested in mouse and their respective positions on human chromosome 5. Arrows mark primer positions used for 3C studies; fixed positions are coloured in red and variable positions in black. (b) Graphical representation of interactions between each enhancer with the differentIrxpromoters, as determined by 3C in two tissues: midbrain/hindbrain (black bars) and limbs (grey bars). The background interaction was calculated as the average of the interactions observed between each fixed position and two regions flanking the promoters. Graphs show means of at least three independent experiments for each enhancer. Asterisks indicate enhancer–promoter interactions that differ significantly from enhancer–control interactions: *P<0.05; **P<0.01; ***P<0.001; Student'st-test. Error bars indicate s.e.m. ExactP-values are listed as follows: 2,260 versusIrx1(brain),P=0.0003; 2,260 versusIrx2(brain),P=0.020; 3,240 versusIrx1(limb),P=0.043; 3,240 versusIrx1(brain),P=0.001; 3,240 versusIrx2(limb),P=0.047; 3,240 versusIrx2(brain),P=0.003; 3,565 versusIrx1(limb),P=0.002; 3,565 versusIrx1(brain),P=0.014; 3,565 versusIrx4(brain),P=0.049; 2,165 versusIrx1(brain),P=0.024; 2,165 versusIrx2(brain),P=0.002. Figure 2: Enhancers physically interact with multiple Irx promoters. ( a ) Expression patterns of the enhancers tested in mouse and their respective positions on human chromosome 5. Arrows mark primer positions used for 3C studies; fixed positions are coloured in red and variable positions in black. ( b ) Graphical representation of interactions between each enhancer with the different Irx promoters, as determined by 3C in two tissues: midbrain/hindbrain (black bars) and limbs (grey bars). The background interaction was calculated as the average of the interactions observed between each fixed position and two regions flanking the promoters. Graphs show means of at least three independent experiments for each enhancer. Asterisks indicate enhancer–promoter interactions that differ significantly from enhancer–control interactions: * P <0.05; ** P <0.01; *** P <0.001; Student's t -test. Error bars indicate s.e.m. Exact P -values are listed as follows: 2,260 versus Irx1 (brain), P =0.0003; 2,260 versus Irx2 (brain), P =0.020; 3,240 versus Irx1 (limb), P =0.043; 3,240 versus Irx1 (brain), P =0.001; 3,240 versus Irx2 (limb), P =0.047; 3,240 versus Irx2 (brain), P =0.003; 3,565 versus Irx1 (limb), P =0.002; 3,565 versus Irx1 (brain), P =0.014; 3,565 versus Irx4 (brain), P =0.049; 2,165 versus Irx1 (brain), P =0.024; 2,165 versus Irx2 (brain), P =0.002. Full size image An evolutionarily conserved 3D architecture of Irx clusters We next evaluated the existence of enhancer–enhancer and promoter–promoter interactions. No interactions were observed between enhancers ( Supplementary Fig. S2a ), but a very strong and significant interaction was detected between the Irx1 and Irx2 promoters ( Fig. 3a ). In contrast, no interactions were found between either of these promoters and the Irx4 promoter ( Fig. 3a and Supplementary Fig. S2b ). Moreover, in contrast to the enhancer–promoter interactions, which were tissue specific, the Irx1 – Irx2 interaction was found in all tissues examined, independently of whether they express these genes (midbrain–hindbrain and E15 limbs, Fig. 3 ) or not (telencephalon and E10 limbs, Supplementary Fig. S3 ). We therefore conclude that this 3D architecture may enable positive or negative coregulation of Irx1 and Irx2 by facilitating equal access of different IrxA enhancers or repressors to their promoters. 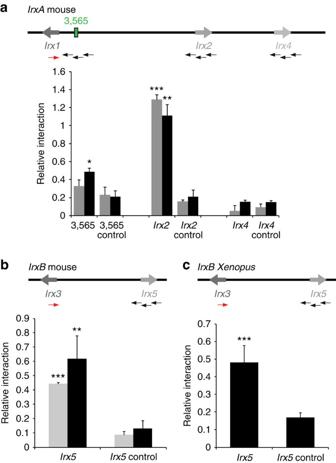Figure 3: An evolutionarily conserved 3D architecture is formed between the first two genes of eachIrxcluster. Arrows show the fixed (red) and variable (black) primer positions used in 3C assays. (a) In mouse tissues, theIrx1promoter strongly and significatly interacts with the 3,565 enhancer and, even more frequently, with theIrx2promoter, but not withIrx4. (b) An equivalent interaction betweenIrx3andIrx5promoters was observed in mouse andXenopusembryos. In these experiments, the fixed primers are situated at theIrx3promoters. Background interaction was calculated, for each species, as the average of the interactions between each fixed position and two flanking regions at a distance of 30 kbp from theIrx5promoters. Graphs show means from at least three independent experiments. Asterisks indicate enhancer–promoter interactions that differ significantly from enhancer–control interactions: *P<0.05; **P<0.01; ***P<0.001; Student'st-test. Error bars indicate s.e.m. ExactP-values are listed as follows:mIrx1versus 3,565 (brain),P=0.023; mouseIrx1versusIrx2(brain),P=0.001; mouseIrx1versusIrx2(limb),P=3.9×10−6; mouseIrx3versusIrx5(brain),P=0.004; mouseIrx3versusIrx5(limb),P=9.2×10−6;Xenopus Irx3versusIrx5,P=2.4×10−4. Figure 3: An evolutionarily conserved 3D architecture is formed between the first two genes of each Irx cluster. Arrows show the fixed (red) and variable (black) primer positions used in 3C assays. ( a ) In mouse tissues, the Irx1 promoter strongly and significatly interacts with the 3,565 enhancer and, even more frequently, with the Irx2 promoter, but not with Irx4 . ( b ) An equivalent interaction between Irx3 and Irx5 promoters was observed in mouse and Xenopus embryos. In these experiments, the fixed primers are situated at the Irx3 promoters. Background interaction was calculated, for each species, as the average of the interactions between each fixed position and two flanking regions at a distance of 30 kbp from the Irx5 promoters. Graphs show means from at least three independent experiments. Asterisks indicate enhancer–promoter interactions that differ significantly from enhancer–control interactions: * P <0.05; ** P <0.01; *** P <0.001; Student's t -test. Error bars indicate s.e.m. Exact P -values are listed as follows: mIrx1 versus 3,565 (brain), P =0.023; mouse Irx1 versus Irx2 (brain), P =0.001; mouse Irx1 versus Irx2 (limb), P =3.9×10 −6 ; mouse Irx3 versus Irx5 (brain), P =0.004; mouse Irx3 versus Irx5 (limb), P =9.2×10 −6 ; Xenopus Irx3 versus Irx5 , P =2.4×10 −4 . Full size image The two vertebrate Irx clusters arose from a genome duplication event that took place at the base of the vertebrate lineage. As a consequence, the overall genomic structure of both clusters is very similar and has been maintained throughout vertebrate evolution. Thus, in all vertebrates, both Irx clusters are very large, the relative distance between genes is similar and there is a conserved orientation of transcripts and distribution of paralogous HCNRs. Moreover, in both clusters, the first two genes are largely coregulated, whereas the third gene shows a more divergent expression pattern (reviewed in ref. 1 ). To test whether the 3D architecture described here, which brings the first two genes of the IrxA cluster into close proximity, is evolutionarily conserved and also forms at the IrxB cluster, we examined the putative interaction between Irx3 and Irx5 , and found that their promoters strongly and significantly interact in both mouse and in Xenopus ( Fig. 3b,c ). Similar to what occurs in the IrxA cluster, no interaction was found between the Irx3 and the Irx6 promoter ( Supplementary Fig. S2c ). By bringing the first two genes of both Irx clusters together, this evolutionarily conserved 3D architecture places them in the same regulatory landscape, probably facilitating similar access by all enhancers. CTCF likely helps form the 3D Irx architecture CTCF is a DNA-binding factor known to facilitate the formation of chromatin loops [20] . To gain insight into the possible implication of CTCF in the physical interaction between Irx promoters, we explored the ENCODE database [21] , available via the UCSC browser [22] , to examine CTCF distribution in different human cell lines. In most human cell lines ( Fig. 4a ), CTCF is bound to the promoters of the Irx genes, preferentially to those of the first two genes of each complex ( Irx1 / Irx2 and Irx3 / Irx5 ). A similar situation occurs in mouse ES and fibroblast cells [23] . This may therefore be an evolutionarily conserved feature of the Irx genes. Accordingly, using the Jaspar and CTCF-binding site databases [24] , [25] , we also found potential CTCF-binding sites in the vicinity of the Xenopus and zebrafish Irx genes ( Supplementary Fig. S4 ). CTCF is therefore a good candidate mediator of the formation of the conserved Irx 3D architecture. To test this possibility, we knocked down CTCF function in zebrafish using two specific morpholinos (see Methods and Supplementary Fig. S5a-c for details). Examination of the contact between the irx3a and irx5a promoters in non-injected (non-morphant) zebrafish embryos revealed a clear and significant interaction ( Fig. 4b ), indicating that the 3D architecture that associates these promoters is also conserved in the fish genome. Reduction of CTCF function in morphant embryos of both types significantly reduced the contact between these promoters ( Fig. 4b ), suggesting that CTCF likely participates in the formation of this 3D architecture in all vertebrates. However, we cannot discard the possibility that the reduced contact between the irx3a and irx5a promoters in the CTCF morphant embryos is an indirect consequence of reduced expression of downstream CTCF targets. 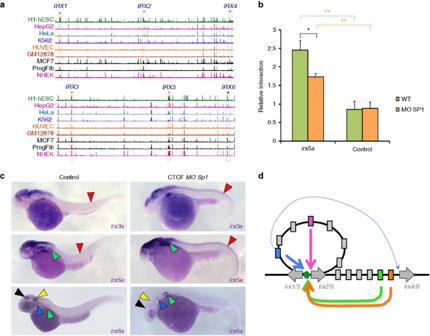Figure 4: The three-dimensionalIrxarchitecture depends on CTCF. (a) Distribution of CTCF binding within theIrxclusters as determined by ChIP-seq in different cell types in the ENCODE project. In most cell types, CTCF is bound to theIrxpromoters (coloured boxes). Note that the first two genes of each complex (orange boxes) are bound by CTCF in more cell types than the promoter of the third gene (grey boxes). (b) 3C assays to detectIrx3andIrx5interactions in zebrafish embryos. The fixed primer is located at theIrx3promoter and the background interaction was calculated as the average of the interactions between the fixed position and two flanking regions at a distance of 30 kbp from theIrx5promoter. A clear interaction is detected between theIrx3andIrx5promoters (green bars), which is significantly reduced in CTCF morphant embryos (orange bars). Graphs show means from at least three independent experiments: *P<0.05; **P<00; Student'st-test. Error bars indicate s.e.m. (c) Expression of zebrafishIrxAagenes in control and CTCF morphant embryos. Note that the levels ofirx3aandirx5aexpression are increased, especially in spinal cord (red arrowheads), whereasirx6ais downregulated in midbrain and hindbrain (black and yellow arrowheads, respectively) and upregulated in the otic vesicle and lateral epidermis (blue and green arrowheads, respectively). (d) Model of the 3D architecture of theIrxclusters. The proximity of the promoters of the first two genes is probably facilitated by CTCF (green circle). Similar access of enhancers to these genes is shown with coloured thick arrows. Restricted access of an enhancer to the third gene of the cluster is shown by the discontinuous thin blue arrow. Coloured boxes: relative positions of the enhancers analysed by 3C. Grey boxes: relative positions of other enhancers identified in this study. Figure 4: The three-dimensional Irx architecture depends on CTCF. ( a ) Distribution of CTCF binding within the Irx clusters as determined by ChIP-seq in different cell types in the ENCODE project. In most cell types, CTCF is bound to the Irx promoters (coloured boxes). Note that the first two genes of each complex (orange boxes) are bound by CTCF in more cell types than the promoter of the third gene (grey boxes). ( b ) 3C assays to detect Irx3 and Irx5 interactions in zebrafish embryos. The fixed primer is located at the Irx3 promoter and the background interaction was calculated as the average of the interactions between the fixed position and two flanking regions at a distance of 30 kbp from the Irx5 promoter. A clear interaction is detected between the Irx3 and Irx5 promoters (green bars), which is significantly reduced in CTCF morphant embryos (orange bars). Graphs show means from at least three independent experiments: * P <0.05; ** P <00; Student's t -test. Error bars indicate s.e.m. ( c ) Expression of zebrafish IrxAa genes in control and CTCF morphant embryos. Note that the levels of irx3a and irx5a expression are increased, especially in spinal cord (red arrowheads), whereas irx6a is downregulated in midbrain and hindbrain (black and yellow arrowheads, respectively) and upregulated in the otic vesicle and lateral epidermis (blue and green arrowheads, respectively). ( d ) Model of the 3D architecture of the Irx clusters. The proximity of the promoters of the first two genes is probably facilitated by CTCF (green circle). Similar access of enhancers to these genes is shown with coloured thick arrows. Restricted access of an enhancer to the third gene of the cluster is shown by the discontinuous thin blue arrow. Coloured boxes: relative positions of the enhancers analysed by 3C. Grey boxes: relative positions of other enhancers identified in this study. Full size image The 3D architecture of the Irx cluster, likely facilitated by CTCF, may serve two functions. First, by bringing together the promoters of the first two genes of the clusters, it might make both genes similarly accessible to most cis -regulatory elements, thus contributing to their coregulation. Second, it might generate a more divergent regulatory landscape for the third gene of the cluster, by reducing the ability of some cis -regulatory elements within the loop to function on the promoter of the third gene. We therefore expect that CTCF impairment should have an impact on the expression patterns of all three genes in the cluster, and this is what we saw in the zebrafish IrxBa cluster in embryos injected with either of the two CTCF-specific morpholinos ( Fig. 4c ). Both irx3a and irx5a were overexpressed all along the neural tube, especially in the spinal cord, and irx6a was downregulated in the midbrain and hindbrain, whereas its expression increased in the otic vesicle and in the lateral epidermis ( Fig. 4c ). Interestingly, these two last domains correspond to tissues expressing one or both of the other irx genes, suggesting that, in the morphants, some enhancers that normally preferentially function on these other genes are now able to efficiently activate irx6a . Our results are therefore compatible with the 3D architecture shown in Figure 4d . Remodelling of the IrxA architecture during teleost evolution If the above model is correct, any disruption of the Irx complexes should have a major impact on the expression of the first two genes, which are coregulated, whereas the third gene, which is present in a more independent regulatory landscape and is controlled by fewer cis -regulatory elements, should be less affected. To test this prediction, we took advantage of a system in which the highly conserved structure of the vertebrate cluster has not been maintained. The genome duplication that occurred at the base of the teleost lineage has provided extra copies of IrxA genes. This permitted divergent evolution [26] , [27] , enabling comparison of the expression of the IrxA genes in clusters with different architectures. In medaka, the IrxAa cluster contains the full set of Irx genes, organized in a manner similar to that of other vertebrates. The expression patterns of medaka IrxAa genes are also similar to those of tetrapod IrxA genes, such as mouse or Xenopus ( Figs 2a and 5a,b ). For example, in medaka and Xenopus , irx1/irx1a and irx2/irx2a are largely coexpressed in broad areas of the neuroectoderm, whereas irx4/irx4a expression is limited to a restricted area of the hindbrain and to the heart ( Fig. 5a,b ). 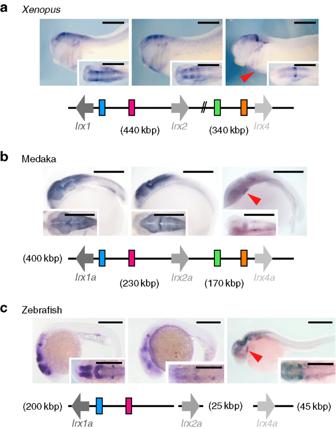Figure 5: Disassembly of theIrxAcluster alters the expression patterns ofIrxAgenes. Genome architecture and expression patterns ofIrxAgenes in (a)Xenopus, (b) medaka and (c) zebrafish. Expression patterns at neurula stages are shown in lateral and dorsal (insets) views. Ina,b, numbers in parentheses indicate the intergenic distances, and incit represents the size of orthologousIrxAaDNA associated with each gene. Red arrowheads point atIrx4expression in the heart. Coloured rectangles: enhancers analysed in this study by 3C. Some of these enhancers, as well as others, were lost upon disaggregation of zebrafishIrxAacluster. Scale bars, 0.5 mm. Figure 5: Disassembly of the IrxA cluster alters the expression patterns of IrxA genes. Genome architecture and expression patterns of IrxA genes in ( a ) Xenopus , ( b ) medaka and ( c ) zebrafish. Expression patterns at neurula stages are shown in lateral and dorsal (insets) views. In a , b , numbers in parentheses indicate the intergenic distances, and in c it represents the size of orthologous IrxAa DNA associated with each gene. Red arrowheads point at Irx4 expression in the heart. Coloured rectangles: enhancers analysed in this study by 3C. Some of these enhancers, as well as others, were lost upon disaggregation of zebrafish IrxAa cluster. Scale bars, 0.5 mm. Full size image In contrast to medaka, the zebrafish IrxAa cluster has split into three ( Fig. 5c ). irx1a remains associated with most of the original Irx1/Irx2 intergenic region (200 kbp) and contains many HCNRs, including those corresponding to the 3,565 and 3,240 enhancers. irx2a and irx4a , on the other hand, retain only 25 and 45 kbp, respectively, from the original cluster sequences, with very few associated HCNRs. The expression of zebrafish irx1a is more restricted than that of the medaka irx1a or irx2a genes ( Fig. 5b,c ). Specifically, zebrafish irx1a is only weakly expressed in the posterior hindbrain and spinal cord. This is in agreement with the reduced number of HCNRs associated with irx1a in zebrafish and with the fact that most hindbrain and spinal cord enhancers identified in this study are located in the intergenic territory between Irx2 and Irx4 . Because of the chromosomal rearrangement in zebrafish, this territory is no longer associated with these genes. The expression of zebrafish irx2a is restricted to only a few domains ( Fig. 5c ), again correlating with the low number of HCNRs associated with this gene. irx4a is expressed in the hindbrain and in the heart ( Fig. 5b,c ), in a manner similar to medaka irx4a , which would indicate that most irx4a enhancers remain associated with this gene in zebrafish. The expression patterns of zebrafish IrxAa genes are therefore compatible with our predictions based on the architectural features of the Irx clusters, namely, that the disruption of the IrxAa cluster in zebrafish has had a major impact on irx1a and irx2a expression, but much less of an effect on irx4a . Developmental genes are expressed in a variety of tissues and at different embryonic stages, fulfilling multiple functions in different processes. To achieve this, their rate of transcription is controlled by multiple cis -regulatory elements, some of them functioning over very long distances [28] , [29] . Our analysis has identified a large number of cis -regulatory elements, located in HCNRs and distributed throughout the 2-Mbp IrxA cluster, and that altogether appear to recapitulate the expression patterns of IrxA genes. Most enhancers drive expression in territories expressing more than one Irx gene, making it likely that different genes of the cluster are regulated in concert. Sharing of cis -regulatory elements between neighbouring genes has often been suggested, but only demonstrated in a handful of cases [30] , [31] , [32] , [33] , [34] . In all these examples, a single enhancer or a locus control region interacts with multiple genes. Using 3C (ref. 19 ), we show that cis -regulatory elements located throughout the IrxA cluster physically interact with more than one Irx promoter, even over distances of 1.6 Mbp (which, to the best of our knowledge, is the most distant physical interaction between an enhancer and a promoter so far reported). Interestingly, the interactions of each enhancer with the promoters seem to occur one by one, as we could not detect interactions between different enhancers. We propose that the presence of shared enhancers is probably the major evolutionary constraint that maintains the association of the Irx genes in clusters. Despite the sharing of enhancers, the expression patterns of all the Irx genes do not completely overlap; the first two genes of both Irx clusters are coexpressed in most tissues, but the third gene shows a more limited and divergent expression pattern [3] , [7] , [11] , [12] , [13] , [14] , [35] , [36] , [37] . Accordingly, we find that enhancers preferentially interact with the two first genes of the IrxA cluster. This raises the important question of how this differential regulation takes place. We demonstrate the existence of a conserved 3D architecture in the Irx clusters, probably dependent on CTCF, which helps to explain this differential regulation. This 3D conformation, which seems to be independent of transcription, brings the promoters of the first two genes of each cluster into close proximity. This would place these genes in the same regulatory landscape, thereby probably facilitating their coregulation, both positive and negative. Moreover, the same 3D architecture would be likely to trap cis -regulatory elements and thus reduce their access to the promoter of the third gene of the complex ( Fig. 4d ), generating a rather different regulatory landscape for this gene. If this model is correct, disruption of the cluster would more strongly affect the expression of the first two genes. This prediction is borne out by the naturally occurred genomic dispersion of the IrxAa cluster in zebrafish. However, definitive demonstration of this model would require the targeted rearrangement of the existing Irx clusters in a model system such as mouse. In several aspects, the Irx genes resemble the Hox genes. Both types of genes encode homeoproteins that are essential for animal development, both are organized in clusters, genes within these clusters share regulatory elements, and the clusters form complex 3D architectures that are probably CTCF dependent [1] , [38] , [39] , [40] . However, despite these similarities, there are also important differences. During evolution, the original Hox cluster appears to have arisen before the arthropod–vertebrate split [38] . In contrast, Irx clusters seem to have arisen independently several times during evolution [2] , [6] . Therefore, in contrast to Hox clusters, clustering of Irx genes in different lineages are not related. Once generated, both these clusters are probably maintained by the use of shared regulatory elements. In Hox clusters, shared regulation is mainly mediated by global control regions that lie outside the clusters [39] . In the Irx clusters, we find many and diverse shared enhancers within the clusters. Nevertheless, we cannot exclude the possibility that other shared Irx enhancers lie outside these clusters. Finally, in Hox clusters, multiple loops, probably dependent on CTCF, are present in silent clusters. These loops are released upon cluster activation, suggesting that they may be associated with the process of cluster silencing. This contrasts with our results, which suggest that contact between promoters in the Irx clusters occurs in a similar manner in tissues independently of whether they express Irx genes, probably facilitating either their coactivation or their corepression. Moreover, our data show that the architecture of the two paralogous clusters is similar, whereas the architecture of the various human paralogous HOX clusters appears to be specific in each case [40] . Finally, it remains to be shown whether, as we show for the Irx clusters, the 3D architecture of orthologous Hox cluster is conserved. On the basis of our findings, we propose that the formation of internal loops in gene clusters, which may be regulated in time and space, would facilitate the formation of specific regulatory landscapes for certain genes of the cluster in a tissue- and stage-dependent manner. This may favour the further sub-functionalization of these independently regulated genes. Thus, the presence of loops may have evolved in these clusters as a new dimension to satisfy a requirement for differential expression of otherwise coregulated genes organized in a linear arrangement in the genome. Animal transgenesis All HCNRs were amplified by PCR from mouse, Xenopus tropicalis or zebrafish genomes using the primers listed in Supplementary Table S1 . The PCR fragments were subcloned in PCR8/GW/TOPO vector and, using Gateway technology, transferred to the corresponding destination vectors for transgenesis in mouse, Xenopus tropicalis or zebrafish. For the generation of transgenic mice, the genomic fragments were transferred into a vector containing the human minimal β-globin promoter, lacZ and a SV40 polyadenylation signal [41] . Vectors were subsequently linearized, the vector backbone removed and the construct microinjected into one-cell mouse embryos. F0 embryos at stages 11.5–13 d.p.c. were collected and stained for lacZ activity. An enhancer was considered positive when three or more independent transgenic embryos showed the same expression pattern. For the generation of transgenic Xenopus , the fragments were transferred into a vector containing the Xenopus 0.6-kbp Gata2 minimal promoter driving green fluorecent protein (GFP) [42] . Transgenesis was performed using the I-SceI method following the protocol already described [43] . Briefly, after in vitro fertilization of the oocytes, one-cell-stage Xenopus embryos were injected with 5 nl of the injection mix, composed of the construct DNA (final concentration 5 ng μl −1 ), 5 U of I-SceI enzyme (New England Biolabs) and 1X I-SceI buffer. In situ hybridization to detect GFP mRNA was used to identify the transgenic embryos. An enhancer was considered positive when ten or more independent transgenic embryos showed the same expression pattern. For the generation of transgenic zebrafish, the fragments were transferred into the ZED vector [44] . Zebrafish transgenic embryos were generated using the Tol2 transposon/transposase method [45] , with minor modifications. One-cell embryos were injected with a 2-nl volume containing 25 ng μl −1 of transposase mRNA, 20-ng μl −1 phenol/chloroform, purified ZED constructs and 0.05% phenol red. For zebrafish, three or more independent stable transgenic lines were generated for each construct. All animal experiments were conducted following guidelines established and approved by local Government and our Institutional Animal Care and Use Committee, and in accordance with best practices outlined by the European Union. Chromosome conformation capture assays Midbrain, hindbrain and spinal cord (M–H samples), limbs and heart were dissected from E15 mouse embryos and processed to obtain single-cell preparations. For Xenopus and zebrafish, single-cell preparations were prepared from total embryos. A total of 10 7 isolated cells were fixed and lysed, and nuclei were then digested with Hin dIII endonuclease (Roche). DNA was then treated with low concentrations of T4 DNA ligase (Promega) to favour intramolecular ligations. A set of locus-specific primers ( Supplementary Table S2 ) was designed with the online program Primer3 v. 0.4.0 (ref. 46 ), each primer being close to a Hin dIII site flanking a chromosomal site of interest. For mouse and Xenopus 3C experiments, we measured the relative enrichment of each ligation product by semi-quantitative PCR, as described in ref. 20 . Each DNA sample was calibrated so that the PCR products were always in the linear range. Primers next to each enhancer were considered fixed primers, and different interactions were tested using primers close to the promoters. For each interaction, two negative-control primers were designed to target sites ∼ 30 kbp upstream and downstream of the region of interest. PCR products were run on an agarose gel and measured with a Typhoon scanner. For the zebrafish 3C experiments, which required precise quantifications, we followed the quantitative PCR protocol indicated in ref. 47 . In all cases, product values were related to a control composed of bacterial artificial chromosomes (BACs) that encompass all our regions of interest (RP23-127L21, RP23-347L10, RP23-93E17, RP23-52B16 and RP23-131B17 for mouse genome; OAAA043I21 and OAAA098B15 for Xenopus ; and DKEY-103G18 and CH211-25M11 for zebrafish). To compare data from different tissues, PCR values were normalized by means of control primers targeting the Ercc3 gene locus in each species. Statistical analysis Assuming that data is normally distributed, one-tailed t -test was performed to test significance of differences among sample averages. In all tests, we adopted an alpha level of 0.05. Differences were considered significant or highly significant when P -values were situated below 0.05 or 0.01, respectively. Zebrafish morpholino injections Two zebrafish morpholinos to knockdown CTCF function were used. MOatg (5′-CGGCCTCAGTCGGTCCCCCTTCCAT-3′) was designed to target the mRNA region spanning the first ATG, to block its translation. MOsp1 was designed to bind to the acceptor splice site between intron 2 and exon 3 (5′-AGCAAATATCACACACTCACCTTTC-3′). A total of 4 or 15 ng of the MOatg or MOsp1 morpholinos, respectively, were injected into one-cell-stage embryos. Morpholino specificity was evaluated by detecting the levels of CTCF protein in the morphant embryos ( Supplementary Fig. S5a,b ). CTCF was detected with the chick CTCF antibody [48] , which recognizes zebrafish CTCF [49] . Western blots were performed as reported in ref. 49 using the anti-CTCF antibody diluted 1:500. To further examine the inhibitory action of MOsp1 on CTCF mRNA splicing, we designed primers targeting exons 2 and 5 (5′-GGAAGAAGAAATGGCTGAACC-3′ and 5′-GGCATAACTGCACAGACTGC-3′). These primers should amplify a 726-bp band only if the morpholino inhibits correct removal of intron 2; retention of this intron in the mRNA introduces several precocious stop codons ( Supplementary Fig. S5c ). For reverse transcription–PCR, total RNA was extracted at 48 h.p.f. from 25 morphants and control embryos, and amplification was carried out for 30 cycles. How to cite this article: Tena, J. J. et al . An evolutionarily conserved three-dimensional structure in the vertebrate Irx clusters facilitates enhancer sharing and coregulation. Nat. Commun. 2:310 doi: 10.1038/ncomms1301 (2011).